Ultrafast cooling reveals microsecond-scale biomolecular dynamics The temperature-jump technique, in which the sample is rapidly heated by a powerful laser pulse, has been widely used to probe the fast dynamics of folding of proteins and nucleic acids. However, the existing temperature-jump setups tend to involve sophisticated and expensive instrumentation, while providing only modest temperature changes of ~10–15 °C, and the temperature changes are only rapid for heating, but not cooling. Here we present a setup comprising a thermally conductive sapphire substrate with light-absorptive nano-coating, a microfluidic device and a rapidly switched moderate-power infrared laser with the laser beam focused on the nano-coating, enabling heating and cooling of aqueous solutions by ~50 °C on a 1-μs time scale. The setup is used to probe folding and unfolding dynamics of DNA hairpins after direct and inverse temperature jumps, revealing low-pass filter behaviour during periodic temperature variations. Experimental studies of fast dynamics of proteins and nucleic acids depend on techniques to rapidly change physical conditions or chemical composition of the medium. To rapidly exchange the medium, microfluidic devices with tight hydrodynamic focusing of a narrow stream of protein solution in a continuous laminar flow have been used, reaching temporal resolutions as high as ~1 μs [1] , [2] . Microfluidic systems require small sample volumes and are compatible with high-resolution optical microscopy, making them well suited for experiments with fluorescently labelled biomolecules [3] , [4] . Nevertheless, hydrodynamic focusing systems require delicate adjustment and careful measurements of high-speed microscopic flows, complicating their practical application. A widely used technique to change physical conditions is the temperature jump (T-jump) [5] , [6] , [7] . Standard T-jump setups tend to be relatively complex, involving powerful pulsed lasers and special Raman converters. Heating during a T-jump occurs by direct deposition of the energy of a laser pulse into the solution on a nanosecond scale. The heated region cools down by thermal conduction, on a time scale proportional to the square of its diameter. For a typical diameter of ~100 μm, the cooling time is ~10 ms [5] . Hence, studies of ultrafast dynamics with the T-jump technique are limited to processes triggered by heating rather than cooling. Moreover, the typical temperature change achievable with the T-jump technique is relatively small (10–15 °C) [5] , further restricting its functionality. Here we present an experimental setup consisting of a light-absorptive thermally conductive substrate, a microfluidic device and an inexpensive near-infrared laser, enabling heating (T-jump) as well as cooling (inverse T-jump) of aqueous solutions by ~50 °C on a 1-μs time scale ( Fig. 1 ). The setup is used on a confocal fluorescence microscope to monitor conformational changes of two DNA hairpins, one short and one moderate length, after direct and inverse T-jumps (iT-jumps), revealing conformational dynamics with folding and unfolding times as short as 3–4 μs. Experiments at different concentrations of salt in the solution indicate that ionic strength has a strong effect on the folding but not on the unfolding rate of the moderate-length DNA hairpin. The setup also enables a conceptually new type of test, in which square waves of temperature are applied and the amplitude of changes in the conformations of DNA hairpins is measured as a function of frequency of the temperature waves. 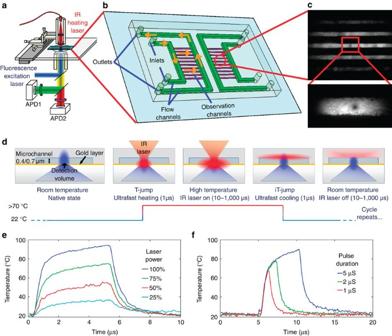Figure 1: Direct and inverse T-jump setup. (a) A moderate-power infrared laser beam is incident from above and focused on the surface of a gold-coated sapphire substrate at the bottom of a 0.4- or 0.7-μm-deep microchannel fabricated in PDMS. Fluorescence imaging is performed on an inverted microscope. (b) Schematic of the microfluidic device used in the experiments. Observation channel depth: 0.4 or 0.7 μm; flow channel depth: 20 μm. (c) Wide-field fluorescence image of the laser-heated spot in a 0.4-μm-deep observation channel filled with HPTS dye taken with a 40X/0.9 objective. (d) Cross-section of an observation channel during a T-jump cycle. (e,f) Temperature as a function of time in the middle of the laser-heated spot in a 0.4-μm-deep channel during a cycle of heating and cooling (average of ~106cycles in each case). Different curves correspond to varying laser powers for 5-μs-long laser pulses (starting at 0.4 μs) (e) and different laser pulse durations with the same power (starting at 5 μs) (f). The temperature is assessed by HPTS fluorescence. Figure 1: Direct and inverse T-jump setup. ( a ) A moderate-power infrared laser beam is incident from above and focused on the surface of a gold-coated sapphire substrate at the bottom of a 0.4- or 0.7-μm-deep microchannel fabricated in PDMS. Fluorescence imaging is performed on an inverted microscope. ( b ) Schematic of the microfluidic device used in the experiments. Observation channel depth: 0.4 or 0.7 μm; flow channel depth: 20 μm. ( c ) Wide-field fluorescence image of the laser-heated spot in a 0.4-μm-deep observation channel filled with HPTS dye taken with a 40X/0.9 objective. ( d ) Cross-section of an observation channel during a T-jump cycle. ( e , f ) Temperature as a function of time in the middle of the laser-heated spot in a 0.4-μm-deep channel during a cycle of heating and cooling (average of ~10 6 cycles in each case). Different curves correspond to varying laser powers for 5-μs-long laser pulses (starting at 0.4 μs) ( e ) and different laser pulse durations with the same power (starting at 5 μs) ( f ). The temperature is assessed by HPTS fluorescence. Full size image The experimental setup The short cooling time is achieved by minimizing the dimensions of the region into which the laser energy is deposited. To this end, we use a microfabricated silicone chip sealed against a thin sapphire substrate with a 20- to 25-nm layer of gold on its surface and focus the beam of a 980-nm infrared laser to a small spot on the substrate. The nanolayer of gold absorbs ~40% of the incident laser power (with ~20% being reflected), thus limiting the lateral and axial dimensions of the heated region to the diameter of the focused beam and the thickness of the gold coating, respectively. The deposition of a large fraction of the laser energy into a microscopically small volume provides high local temperatures with a moderate-power (~160 mW), continuous wave heating laser. Cooling of the heated region is accelerated by the high thermal conductivity of the sapphire substrate, which is ~20 times greater than that of common borosilicate glass (see Methods). To limit the axial extension of the region from which the fluorescence signal is collected, we performed the experiments in microchannels with depths of 0.4 or 0.7 μm. Importantly, unlike the flow-focusing microfluidic devices previously used for protein-folding studies, the folding reaction time is evaluated using optics and electronics only, with measurements performed at a single spot, and without the need for precise control or extensive calibration of the flow. Low-velocity perfusion (10–100 μm s −1 ) is used only to prevent evaporation and excessive photobleaching of the sample. Measurements of temperature The temperature in the microchannels has been evaluated using a pH-sensitive fluorescent dye, 8-hydroxypyrene-1,3,6-trisulfonic acid (HPTS), in 50 mM Tris buffer, whose pH has a strong dependence on the solution temperature. The temperature dependence of HPTS fluorescence has been measured under a fluorescence microscope using a modified version of the microfluidic device and has been found to be nearly linear ( Supplementary Fig. 1 ). The spatial distribution of fluorescence in the 0.4-μm deep microchannel under the infrared laser heating indicates that the heated region has a full width at half maximum of ~3 μm ( Supplementary Fig. 2 ). With the infrared laser periodically switched on and off, with different powers, duty cycles, and periods, under stroboscopic wide-field fluorescence illumination, we have consistently found the iT-jump time, defined as the cooling time to 50% of the initial T-jump (half-decay time), at ~0.45 μs, in good agreement with our numerical simulations. A more conservative estimate of the temperature half-decay time, taking into account the non-uniformity of the temperature in the sampling region before and during an iT-jump, is ~0.80 μs (see Supplementary Note 1 and Supplementary Fig. 5a,b ). In the beginning of a T-jump, the temperature increases nearly linearly in time at a rate proportional to the laser power, reaching ~93 °C μs −1 for the highest power tested ( Fig. 1e and Supplementary Table 1 ). Folding and unfolding dynamics of DNA hairpins To further test the functionality of the setup, we have used it to study the folding and unfolding dynamics of an 8-nucleotide-long single-stranded DNA (ssDNA) hairpin, HP1, which are expected to be rapid [8] . Hairpins are dynamic secondary structural elements of nucleic acids that participate in numerous important biological processes [9] , [10] , [11] . Whereas hairpin folding landscapes have been extensively studied using stopped-flow and T-jump techniques [8] , [12] , [13] , [14] , [15] , [16] , much about their dynamics remains unknown. HP1 is fluorescently labelled with tetramethylrhodamine (TMR; Fig. 2a ), such that in the folded state the dye fluorescence is significantly quenched by a proximal guanosine. The T-jump experiments are performed in 0.7-μm-deep microchannels under a confocal microscope focused at the gold-coated substrate. The iT-jump time is measured at 0.6 μs, in good agreement with numerical simulations. The T-jump is from room temperature, T r =22°C to ~55 °C, well above the melting temperature of HP1 at 600 mM NaCl, T m ≈38 °C. On both direct and inverse T-jumps, the fluorescence of HP1 is detectably different from the fluorescence of a non-hairpin control ( Fig. 2a ). 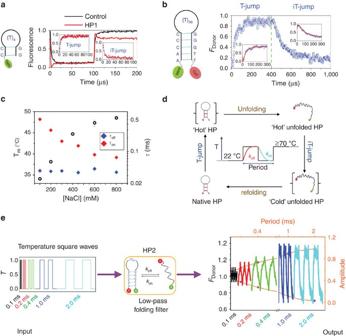Figure 2: Folding and unfolding dynamics of hairpin DNA. Normalized fluorescence of TMR-labelled HP1 (a) and normalized donor fluorescence of Alexa488/Cy5-labelled HP2 (b) as functions of time at 600 mM NaCl. The infrared laser is on/off for 100/100 μs inaand 400/1,600 μs inb. The black line inais the T-jump/iT-jump response of a TMR-tagged non-hairpin ssDNA control. The insets inaandb(same axis labels) show single-exponential fits of the unfolding (left) and refolding (right) data (seeSupplementary Tables 1 and 2). The initial burst phases in the insets inbare the T-jump/iT-jump response of Alexa488 in a hairpin control without the acceptor fluorophore (Supplementary Fig. 10). (c) The effect of [NaCl] on the stability of HP2, as measured byTm(left axis, black circles), and on the relaxation dynamics, as measured byτon/off(1/kon/off;Supplementary Table 3) (right axis, red and blue diamonds). (d) Schematic showing the cyclic occurrence of four states of the hairpins, when square waves of temperature are applied. (e) Dynamic response of HP2 at 200 mM NaCl to square waves of temperature. Temperature waves (input) with periods of 0.1, 0.2, 0.4, 1.0 and 2.0 ms are shown by black, red, green, blue and cyan curves, respectively. Normalized donor fluorescence response (output) during these temperature waves. The orange envelope is the frequency response of HP2 from the model presented inSupplementary Note 2. The data can be fitted with single-exponent kinetics for both T-jump and iT-jump, with time constants of 3.5 and 4.3 μs, respectively ( Supplementary Table 2 ), consistent with an apparent two-state mechanism. When corrected for the finite time of the temperature changes using the numerical simulations, the values of characteristic relaxation times after the T-jump and iT-jump are found at 2.4 and 3.4 μs, respectively, corresponding to unfolding and folding rates ( k − and k + ) of 3.5 × 10 5 and 2.5 × 10 5 s −1 , respectively (see Supplementary Table 2 and Supplementary Fig. 8 ). These rates are in reasonable agreement with the values k − =1.8 × 10 5 s −1 and k + =2.9 × 10 5 s −1 , as previously measured for HP1 at room temperature using fluorescence correlation spectroscopy [8] . The short time scale of the iT-jump and large temperature changes provided by our setup are essential for resolving the kinetics of folding and unfolding of HP1. Figure 2: Folding and unfolding dynamics of hairpin DNA. Normalized fluorescence of TMR-labelled HP1 ( a ) and normalized donor fluorescence of Alexa488/Cy5-labelled HP2 ( b ) as functions of time at 600 mM NaCl. The infrared laser is on/off for 100/100 μs in a and 400/1,600 μs in b . The black line in a is the T-jump/iT-jump response of a TMR-tagged non-hairpin ssDNA control. The insets in a and b (same axis labels) show single-exponential fits of the unfolding (left) and refolding (right) data (see Supplementary Tables 1 and 2 ). The initial burst phases in the insets in b are the T-jump/iT-jump response of Alexa488 in a hairpin control without the acceptor fluorophore ( Supplementary Fig. 10 ). ( c ) The effect of [NaCl] on the stability of HP2, as measured by T m (left axis, black circles), and on the relaxation dynamics, as measured by τ on/off (1/ k on/off ; Supplementary Table 3 ) (right axis, red and blue diamonds). ( d ) Schematic showing the cyclic occurrence of four states of the hairpins, when square waves of temperature are applied. ( e ) Dynamic response of HP2 at 200 mM NaCl to square waves of temperature. Temperature waves (input) with periods of 0.1, 0.2, 0.4, 1.0 and 2.0 ms are shown by black, red, green, blue and cyan curves, respectively. Normalized donor fluorescence response (output) during these temperature waves. The orange envelope is the frequency response of HP2 from the model presented in Supplementary Note 2 . Full size image Next, we have examined a 40-nucleotide ssDNA hairpin, HP2, labelled with a Förster (fluorescence) resonance energy transfer (FRET) dye pair ( Fig. 2b ). In these experiments, the sampling region is heated to ~70 °C, well above T m ≈45 °C for HP2 at 600 mM NaCl. As anticipated, HP2 has slower kinetics than HP1, with relaxation times of 42 and 110 μs during the T-jump and iT-jump, respectively ( Fig. 2b ). Numerical simulations indicate that the diffusion of either HP1 or HP2 into and out of the sampling region during the T-jump/iT-jump experiments has no appreciable effect on the experimental results. We have next probed the effect of NaCl concentration on the folding and unfolding of the DNA hairpins. For HP2, at all tested [NaCl] the calculated folding times at 22 °C and unfolding times at 70 °C are very close to the relaxation times measured in the iT-jump and T-jump experiments, respectively, ( Supplementary Table 3 ). The unfolding time of HP2 at 70 °C remains nearly constant, while its folding time at 22 °C decreases substantially with [NaCl] in the range from 100 to 800 mM, showing an inverse correlation with T m ( Fig. 2c and Supplementary Table 3 ). This result suggests that increased ionic strength has similar stabilizing effects on the folded hairpin and the transition state, but not on the unfolded ssDNA, leading to a significant [NaCl] dependence for folding but not unfolding. The considerable increase of the HP2 folding rate with [NaCl] at 22 °C and the near lack of dependence of the HP2 unfolding rate on [NaCl] at 70 °C are both in agreement with what was found for a similar hairpin [17] . In addition, the rates of HP2 unfolding and folding at 100 mM NaCl and 22 °C, 0.13 × 10 3 and 1.7 × 10 3 s −1 ( Supplementary Table 3 ), agree reasonably well with previously measured values for that hairpin (~0.4 × 10 3 and 4.0 × 10 3 s −1 ) [17] . For HP1, there is no substantial difference in the hairpin stability and in either folding or unfolding rates between [NaCl] of 100 and 600 mM ( Supplementary Table 2 ). This difference between the dependence of HP1 and HP2 folding parameters on [NaCl] can be attributed to Na + -dependent loop stability, as previously proposed [18] , because HP2 has a significantly larger loop size than HP1. Finally, we have tested the dynamic response of HP2 to temperature periodically varying between 22 and 70 °C in a square wave with equal on and off times, and with frequencies ranging from 1,000 to 20,000 Hz. At low frequencies, complete folding and unfolding transitions are observed, as evidenced by full amplitudes of variation in FRET. However, as the frequency is increased ( Fig. 2e ), the amplitude of FRET variations gradually decreases, consistent with a model in which HP2 molecules do not have sufficient time to fully unfold and refold within a period of the temperature wave ( Supplementary Note 2 ). Therefore, the folding of HP2 responds to temperature variations similar to low-pass filters in electronics and cellular signalling networks [19] , [20] , [21] . However, in contrast to electronic low-pass filters, the folding and unfolding times of HP2 are not equal. As a result, the frequency response of HP2 mostly depends on the folding transition, which has a longer time scale ( Supplementary Note 2 and Supplementary Fig. 12 ). Whereas the folding dynamics of proteins and nucleic acids after one–off changes in temperature or medium composition can be studied with the existing techniques, our setup enables studies of folding when the medium conditions have a complex temporal pattern. We present an experimental setup enabling cooling (iT-jump) on a 1-μs time scale, several orders of magnitude faster than with existing T-jump systems. The setup uses an inexpensive, moderate-power infrared laser, which is switched on and off with a home-made driver. The setup is based on a simple and easy-to-operate microfluidic device and does not require fine-tuning or careful calibration of flow rates for accurate evaluation of the folding reaction time. The large range of temperature variation provided by the setup (>70 °C) makes it potentially applicable to probing the folding of a wide variety of proteins and nucleic acids under native medium conditions. The setup is applied to study the rapid dynamics of folding and unfolding of DNA hairpins in solutions with different ionic strengths. Another novel functionality of the presented setup is the periodic variations of temperature with different amplitudes, frequencies and duty cycles, which may reveal hidden features in the folding landscapes of proteins and nucleic acids. Microfluidic setup The microfluidic device consists of a microfabricated polydimethylsiloxane (PDMS) chip and an ~0.15-mm-thick gold-coated sapphire coverslip. Cooling of the heated region is accelerated by the high thermal conductivity of the sapphire substrate, which is ~20 times greater than that of common borosilicate glass ( http://www.mateck.com/index.php?option=com_content&view=article&id=66&Itemid=21 ). The PDMS chip is cast using a photolithographically fabricated master mould and has channels of two different depths, 20 and 0.7 μm (or 0.4 μm). To make the master mould, a silicon wafer is spin-coated with a 0.7 (or 0.4)-μm layer of an ultraviolet-curable epoxy (SU8 by MicroChem, Newton, MA), exposed to ultraviolet light through a photomask, spin-coated with a 20-μm layer of the SU8 epoxy, exposed to ultraviolet light through another photomask and, finally, baked and developed. The microfluidic device has two mirror-symmetric channel networks. Each network has two 20-μm-deep perfusion channels with widths between 200 and 300 μm, each connecting an inlet and an outlet, and an array of parallel, 0.75-mm-long, 10-μm-wide and 0.7 (or 0.4)-μm-deep observation channels between parallel segments of the perfusion channels ( Supplementary Fig. 1a ). The T-jump and iT-jump experiments were performed in the shallow observation channels. The relatively deep perfusion channels are used to rapidly fill the observation channels with solutions of fluorescent dyes and biomolecules, and to maintain a continuous, low-speed perfusion through the observation channels to prevent excessive photobleaching and drying (caused by evaporation through porous PDMS). After all channels in the channel network on the left are filled, inlet 2 and outlet 1 are blocked and the pressure at inlet 1 is set at ~1.0 kPa above the pressure at outlet 2, thus providing a continuous perfusion through the observation channels at a mean flow velocity of ~20 and ~50 μm s −1 in 0.4- and 0.7-μm-deep observation channels, respectively. (The differential pressure of 1.0 kPa is set by placing the solution in the reservoir connected to inlet 1 at ~100 mm above the solution at the reservoir connected to outlet 2.) The two mirror-symmetric copies of the channel network present in the device make it possible to test the dynamics of cooling and heating during T-jumps with temperature-sensitive fluorescent dye (HPTS in Tris buffer) at the same conditions as in the experiments on fluorescently labelled DNA hairpins. The devices with 0.7-μm-deep observation channels are made from Sylgard 184 silicone elastomer (by Dow Corning). As microchannels made of Sylgard 184 are prone to spontaneous collapse when their depth is <0.6 μm, the 0.4-μm-deep observation channels are fabricated in a harder version of PDMS (hPDMS). To prepare hPDMS prepolymer, first, vinyl-substituted PDMS (VDT-731; Gelest, Morrisville, PA) is mixed with 35 p.p.m. platinum catalyst (platinum-divinyltetramethyldisiloxane complex in xylene; Gelest) and 0.25% modulator (2,4,6,8-tetramethyltetravinylcyclotetrasiloxane; Fluka Chemie, Switzerland) is added to it. It is then mixed with hydrogen-substituted PDMS (HMS-301; Gelest) in a 3.4:1 ratio. As hPDMS has poor mechanical properties and readily cracks when bent or perforated, a piece of hPDMS with 0.4-μm channels on its surface is imbedded in a tougher Sylgard 184 matrix. To this end, droplets of hPDMS prepolymer are dispensed onto regions of the master mould with the 0.4-μm-tall relief and partially cured, making soft, dome-shaped solid structures. An ~3-mm layer of Sylgard 184 PDMS prepolymer is then poured onto the master mould and partially cured (to make a soft solid as well). The composite hPDMS–PDMS layer is separated from the mould, cut into individual chips, and the inlet and outlet holes are punched in the chips using blunt Luer needles. The chips are hard baked to completely cure the silicones and are subsequently bonded to the gold-coated sapphire coverslip substrates by overnight baking at 80 °C in an oven. The coating of the sapphire coverslips with an ~20-nm layer of gold is performed on a sputtering machine (Discovery 18, Denton Vacuum) using a standard protocol with a 5-nm priming layer of titanium. The design of the DNA hairpins The temperature-dependent conformational dynamics of two DNA hairpins with distinct folding properties, HP1 and HP2, have been investigated in this study. HP1 is an 8-nucleotide-long ssDNA with complimentary CC and GG sequences on its 5′- and 3′-end, respectively, forming the stem of the hairpin, and TTTT in the middle, forming the loop ( Fig. 2a ). The 5′-end of HP1 is labelled with a TMR fluorophore, whose fluorescence is quenched in the folded state by an adjacent guanosine nucleotide in the 3′-end [22] . The quenching provides an effective means of monitoring the conformation of HP1 by recording the fluorescence intensity of the TMR dye. HP2 is a 40-nucleotide-long ssDNA, 5′-AACCC-(T) 30 -GGGTT-3′, which has 5-nucleotide-long complimentary sequences on its ends. The 5′-end of HP2 is labelled with Alexa488 dye (FRET donor) and the 3′-end is labelled with Cy5 dye (FRET acceptor). As a result, the folded state has maximal FRET efficiency and minimal donor fluorescence, while the reverse is true for the unfolded state. In our experiments, we monitor the conformation of HP2 by measuring the intensity of fluorescence of Alexa488, with Cy5 dye playing the role of a quencher that is active in the folded state (akin to the quenching of TMR dye by guanosine in HP1). To distinguish between changes in the dye fluorescence caused by the hairpin folding (and resulting changes in the quenching) and the direct effect of temperature on the fluorescence of the fluorophores attached to ssDNA, the following DNA constructs are used as negative controls: 5′-TMR-CCTTTT-3′ for HP1 and 5′-amino modifier (C6)-AACCC-(T) 30 -GGGTT-Cy5-3′ and 5′-Alexa488-AACCC-(T) 30 -GGGTT-3′ for HP2. Preparation of the DNA hairpins All of the HPLC-grade synthetic oligonucleotides have been purchased from IDT (San Diego, CA) and used as received, unless otherwise stated. The sequences for HP1 and HP2 are 5′-TMR-CCTTTTGG-3′ and 5′-Alexa488-AACCC-(T) 30 -GGGTT-Cy5-3′, respectively. HP1 has been purchased with TMR dye at the 5′-end. For HP2, the purchased sequence contains a 5′-amino modifier (C6) and a 3′-Cy5 fluorophore. The 5′-end of the ssDNA is labelled with Alexa488 by coupling the amino group with the N-hydroxysuccinimidyl ester of the dye (Alexa488-NHS ester, Molecular Probes). The labelling reaction is carried out in a freshly prepared 100-mM bicarbonate buffer (pH 8.9). The DNA to dye molar ratio is 1:50 and the reaction mixture is incubated overnight in the dark at room temperature. The labelled DNA is separated from unreacted dye by multiple ethanol precipitations. Absorption measurements show >90% labelling efficiency. As Alexa488 serves as the donor in the resulting FRET pair, this degree of labelling has been deemed satisfactory and no further purification steps have been performed. The 5′-Alexa488-AACCC-(T) 30 -GGGTT-3′-negative control has been purchased with the 5′-amino modifier (C6) and labelled with Alexa488 as HP2. Bulk fluorescence measurements Bulk fluorescence measurements have been performed in an ISS fluorimeter, equipped with a Peltier-type temperature controller. DNA concentrations of 200 nM in 10 mM phosphate buffer (pH 7.4) are used for all of the experiments. Excitation wavelengths of 547 nm for TMR (HP1) or 470 nm for Alexa488 (HP2) are used, and the fluorescence intensities at 565 and 518 nm are measured for HP1 and HP2, respectively. To determine the melting temperatures, T m , of the hairpins, the fluorescence of either TMR (HP1) or Alexa488 (HP2) is recorded in a temperature range of 10–75 °C with 2–5 °C intervals. To probe the effect of salt concentration on T m , the following [NaCl] are used: 100 and 600 mM for HP1 and 100, 200, 400, 600 and 800 mM for HP2. The tests are repeated for the three negative controls (see above) to evaluate the inherent (not folding-specific) temperature dependences of fluorescence of the ssDNA-bound fluorophores at each [NaCl]. The fluorescence of the negative controls is fitted with a third-order polynomial of temperature (A+B 1 T+B 2 T 2 +B 3 T 3 ). The fits are then used to obtain corrected melting curves of the two hairpins. The corrected melting curves are fitted using a two-state model with the midpoint of the transitions corresponding to the melting temperatures, T m . Optical setup For local heating of the gold nanolayer on the sapphire substrate, we use a 160-mW, single-mode, fibre-coupled, 980-nm continuous wave infrared laser (Nortel LC92JG74-20). The laser is powered by a home-built driver, making it possible to adjust the power of the laser and switch it on and off on a time scale of ~0.1 μs. The laser light is collimated using an achromatic lens with a focal length of 30 mm and focused using an aspheric lens with focal length of 8 and numerical aperture of 0.50, both of which are assembled inside a tube (all parts by Thorlabs). The assembly is mounted on an XYZ translational stage (Newport), which is attached to the frame on an inverted fluorescence microscope. We note that aqueous solutions in microchannels can also be directly heated using an infrared laser with a wavelength of ~1,455 nm, where water has a relatively strong absorption, with an attenuation length of 305 μm [23] . Nevertheless, the direct heating approach becomes increasingly impractical for shallow channels, with only ~0.13 and 0.23% of light absorbed in 0.4- and 0.7-μm-deep channels, respectively, requiring very powerful lasers and potentially making the heating less localized along the z -axis because of the residual absorption of the infrared light in PDMS. The gold nanolayer coating used in the present study absorbs >2 orders of magnitude greater part of the light (~40%), thus making it possible to use moderate-power infrared lasers with a range of wavelengths. Moreover, the use of the gold nanolayer minimizes the z -axis dimension of the heated region. The experiments on the visualization of the hot spot and rapid cooling (iT-jump) in 0.4-μm-deep observation channels are performed on a Nikon TE300 microscope under widefield fluorescence illumination. The illumination is provided by a high-power 455-nm light-emitting diode (LED; CBT-40 by Luminous Devices), which is mounted in a modified Nikon fluorescence lamp house and powered by another home-built driver that enables switching the LED on and off on an ~0.1-μs time scale. Both drivers are controlled via a National Instruments PCI-6111 Data Acquisition computer interface card, with a LabView (National Instruments) code. Fluorescence images are taken with a fluorescein isothiocyanate filter set, 40X/0.90 Nikon objective and cooled CCD Camera (Cooke SensiCam QE). To visualize fluorescence of the HPTS dye in the observation channel at a certain interval after the infrared laser is switched on or off, stroboscopic fluorescence illumination is used. The infrared laser is pulsed with a controlled duty cycle and period, τ . The fluorescence illumination is phase locked with respect to the infrared pulsing and switched on for Δt =100–200 ns at a time, with a temporal resolution of 100 ns, using the Data Acquisition computer interface card and the LabView code. The exposure time of the camera is set to a value, t cam (typically, 1–10 s), corresponding to ~10 6 periods of infrared pulsing, such that the cumulative time of the fluorescence illumination, t cam · Δt / τ , provides sufficient fluorescence signal. With this imaging technique, every micrograph shows the distribution of fluorescence within a time window Δt at a certain time point, t , of the infrared laser pulsing cycle. The micrographs are taken with values of t covering the entire period of the infrared laser cycle to obtain the intensity of fluorescence in the central 0.8-μm diameter area of the laser-heated spot as a function of time, t . The calibration of the intensity of fluorescence of HPTS as a function of temperature (see below) is then used to plot the apparent temperature in the centre of the laser-heated spot as a function of time, t , during the laser-heating cycles ( Fig. 1e,f ). Temperature calibration To measure the local temperature in an observation channel, we have filled the device with a 100-p.p.m. solution of HPTS in 50 mM Tris buffer, pH=7.5, at room temperature (22 °C). The intensity of HPTS fluorescence is a rapidly increasing function of pH of the solution. As the temperature increases, pH of the Tris buffer decreases, leading to ~2-fold reduction of the HPTS fluorescence, as the temperature is raised from 20 to 80 °C ( Supplementary Fig. 1b ). To obtain the dependence of HPTS fluorescence on temperature in an observation channel, we have used a modified version of the T-jump microfluidic device, which has a PDMS chip with two layers of channels ( Supplementary Fig. 1a ). The first layer of channels engraved on the surface of PDMS is the same as in the T-jump microfluidic device with 0.7-μm-deep observation channels. The second layer consists of a single water-circulation channel with a depth of 2.5 mm, width of 4.2 mm and a length of 14 mm, which is positioned above the array of observation channels, with its bottom 160 μm above the surface of the PDMS chip. The PDMS chip is sealed against a standard 1.5 microscope cover glass, the first-layer channels are filled with the 100-p.p.m. solution of HPTS in Tris buffer and the water-circulation channel is connected to a commercial circulating water bath (Fisher Scientific 9101). The water circulation tubing consists of two long (~1 m) thermally insulated segments with internal diameter (ID) of 1/4", which are connected to the inlet and outlet of the circulating bath, and short (~10 cm) segments of tubing with ID=1/16" connecting the 1/4" tubing and the microfluidic device [24] . The flow rate of the temperature-controlled water through the microfluidic device is measured at a high value of ~2.5 ml s −1 , suggesting that the heat losses by thermal conductivity through the microfluidic device have minimal effect on the temperature of water in the circulation channel. Two calibrated thermistors are inserted into the 1/4′′ ID tubing segments at equal distances upstream and downstream of the microfluidic device and the temperature in the circulation channel, T c , is evaluated as the average of the temperature readings from the two thermistors [24] . The difference between the temperature readings of the two thermistors has followed a trend of being ~1% of the difference between their mean temperature and room temperature. The intensity of fluorescence of HPTS is measured using the same light source (455 nm LED), filter set (fluorescein isothiocyanate) and objective (Nikon 40X/0.90) as in the T-jump experiments. The distance between the cover glass and the front lens of the objective is ~0.50 mm. Given the thicknesses and thermal conductivities of the layers of PDMS between the circulation and observation channels, and of air between the objective and the cover glass (160 μm and 0.15 W m −1 ; 0.5 mm and 0.025 W/m, respectively), as well as the thickness and thermal conductivity of the cover glass (170 μm and 1.0 W m −1 ), we estimate the temperature in the observation channel, T t , as , where T r =22 °C is the temperature of the front lens, which is assumed to be equal to the room temperature. By varying the temperature in the circulator from 20 to 80 °C, we have found that the HPTS fluorescence intensity, I , decreases nearly linearly with T t ( Supplementary Fig. 1b ). A linear fit to the data is made and the resulting linear calibration curve, I versus T t , is used to obtain the local temperature from the local fluorescence intensity in the T-jump/iT-jump experiments. Importantly, the use of the same temperature-sensitive fluorescent solution (100 p.p.m. of HPTS in Tris), same optical setup and observation channels with similar depths (0.7 μm versus 0.4 or 0.7 μm) reduces to a minimum the experimental uncertainly in the application of the calibration curve to the T-jump/iT-jump experiments ( Fig. 1e, f ; Supplementary Figs 5, 9 and 11 ). Measurements of hairpin dynamics in the iT-jump setup The fluorescence of the donor dyes attached to the DNA hairpins and respective controls (TMR for HP1 and Alexa488 for HP2) as a function of time during T-jumps and iT-jumps in the microfluidic device has been measured on a confocal setup (described in detail elsewhere [25] ) with the Olympus 40X/0.90 objective lens. The observation channels in these experiments have a depth of 0.7 μm. The increased depth makes the microfluidic device easier to work with, while still providing a very short cooling time (0.6 μs half-decay time as compared with 0.45 μs for the 0.4-μm channel; see Supplementary Fig. 5 and Supplementary Note 1 ). The dynamics of temperature in the sampling volume during T-jumps/iT-jumps is measured using the same confocal setup, with the 100 p.p.m. solution of HPTS in 50 mM Tris buffer in the observation channel (see Supplementary Figs 4 and 5 , and the Supplementary Note 1 for further details). All fluorescently labelled ssDNA samples are at a concentration 1 μM in 10 mM phosphate buffer (pH 7.4). The fluorescence illumination is derived from a 543-AP-A01 tunable argon-ion laser (Melles-Griot, Carlsbad, CA), with the 514-and 488 nm lines used for TMR and Alexa488, respectively. The collected fluorescent light is detected by an avalanche photodiode (SPCM-AQR-14; Perkin-Elmer, Fremont, CA) with a time resolution of 100 ns. In the T-jump/iT-jump experiments on HP1 (and its negative control), the infrared laser is switched on (at ~100 mW) and off periodically, with both on and off times equal to 100 μs. The infrared laser heating/cooling cycle is typically repeated ~50,000 times (~10 s) and the collected fluorescence signal is binned into 0.1–1.0 μs intervals within the 200 μs period. The time point when the infrared laser is switched on serves as the reference point within each cycle. To reach a satisfactory signal/noise ratio, the cycling is typically repeated 50 times (2.5 × 10 6 periods; ~10 min total). For HP2 (and its negative control), the infrared laser pulse is on for 400 μs and off for either 1,600 or 9,600 μs, resulting in 2 or 10 ms periods. The binning intervals are 1–10 μs. To reach a satisfactory signal/noise ratio, there are typically 50 temperature cycling series with 10,000 heating/cooling cycles in each (0.5 × 10 6 periods; ~20–100 min total). In the experiments on the dynamic response of HP2 to square waves of temperature, we have varied the period of the infrared laser on/off cycles (temperature wave) from 100 to 2,000 μs, with the on and off times always equal to each other (and to one half of the period). How to cite this article : Polinkovsky, M. E. et al. Ultrafast cooling reveals microsecond-scale biomolecular dynamics. Nat. Commun. 5:5737 doi: 10.1038/ncomms6737 (2014).